Atom manipulation on an insulating surface at room temperature Atomic manipulation enables us to fabricate a unique structure at the atomic scale. So far, many atomic manipulations have been reported on conductive surfaces, mainly at low temperature with scanning tunnelling microscopy, but atomic manipulation on an insulator at room temperature is still a long-standing challenge. Here we present a systematic atomic manipulation on an insulating surface by advanced atomic force microscopy, enabling construction of complex patterns such as a ‘Swiss cross’ of substitutional bromine ions in the sodium chloride surface. Ever since the first systematic atomic manipulation of xenon on a nickel surface at low temperature with scanning tunnelling microscopy in 1990 (refs 1 , 2 ), we have been able to directly control surface structures. By moving and positioning single atoms to certain atomic sites, controlled quantum phenomena can be measured [3] , [4] , [5] . Single chemical reactions of molecules instigated by a local probe have also been reported [6] , [7] , [8] , [9] , [10] . Further, atomic-scale logic devices have been designed, fabricated and operated [11] , [12] , [13] , [14] . The ultimate aim of such studies is next-generation atomic-scale electro-mechanical devices [15] , operating at room temperature (RT) on a dielectric substrate. There are two characteristic classes of atom and molecule manipulations: mechanical- and electron-induced manipulations. In mechanical-induced manipulation, the attractive and repulsive interaction forces between the probe tip and the target object are used to drive the motion [16] , [17] , [18] , [19] , [20] . In contrast, in electron-induced manipulation the atom or molecule is excited by the inelastic tunnelling electron and hence they start to diffuse themselves [21] , [22] , [23] , [24] . In both modes, manipulation at RT requires a delicate balance between a high enough initial binding energy to the substrate to avoid desorption and a small enough diffusion barrier to be able to be influenced by the local probe tip. Owing to the large binding energy of molecule to metal surfaces, such molecule manipulations have already been reported in the mid-nineties [25] , [26] . Systematic atomic manipulation at RT was successfully conducted on semiconductor surfaces where strong, directional covalent bondings of Si, Ge, Sn and Pb give rise to reconstructions of the surface [17] , [20] , [27] . In those experiments, atomic interchange manipulation among group 4 semiconductors were used to move the atom in vertical and lateral directions. On a fully insulating surface, the restriction to mechanical manipulation via atomic force microscopy (AFM) [28] , and the smaller diffusion barrier of adsorbed species [29] make this task particularly challenging. Several attempts were recently conducted, but the manipulation mechanisms were not controllable enough to precisely achieve the desired results [30] . Thus, fabrication of artificial structures on an insulator is still a long-standing challenge, even at low temperature. In this article, we present the first systematic atomic manipulation on an insulating NaCl(001) surface under ultra-high vacuum (UHV) conditions at RT. Bimodal dynamic mode AFM We use the recently developed bimodal dynamic mode AFM (bimodal d-AFM) [31] , [32] , [33] , in which the vertical and lateral tip–sample interactions are simultaneously detected via frequency shifts of the flexural Δ f ver and torsional resonance modes Δ f TR , respectively [34] . In this technique, the Δ f TR signal has extreme sensitivity to the atomic-scale interaction, and hence atomic resolution is reliably achieved in a wide range of the Z tip–sample distance. This advantage is beneficial for atomic manipulation, in which the interaction force is used both for imaging and manipulation, depending on the magnitude in a controlled manner. The tip apex of a Si cantilever was terminated with NaCl by prior indentation to the sample surface, a standard procedure on insulating substrates [35] . 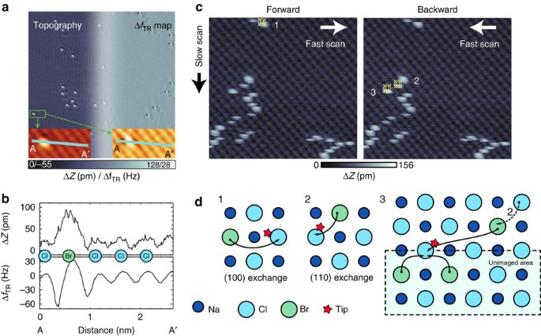Figure 1: Lateral atom manipulations. (a) Topography (left) and torsional frequency shift ΔfTRmap (right) of the sodium chloride (NaCl) surface obtained at second flexural frequency shift Δf2nd=−144 Hz in an area of 28 × 28 nm, and (b) corresponding line profiles along A–A'. (c) Forward and backward topography maps, obtained at Δf2nd=−194 Hz in an area of 8.7 × 8.7 nm, revealing Br−manipulation events. (d) Models of three different types of manipulation deduced from the images inc. Measurement parameters for all images: amplitudes of the second flexural modeA2nd=300 pm and the torsional modeATR=50 pm. Lateral atom manipulations Figure 1a shows the topography (left) and the Δ f TR maps (right) observed in an area of 28 × 28 nm with the bimodal technique, and reveals the typical contrast pattern of NaCl (100) with defects appearing as brighter atomic sites. We can attribute these defects to Br − ions, whose presence in the crystal was confirmed by X-ray fluorescence analysis ( Supplementary Fig. 1 ; Supplementary Table 1 ; and Supplementary Note 1 ). The concentration observed by AFM ( Fig. 1a ) is one order of magnitude higher than this bulk measurement, and the increase of the population is most probably due to the segregation of Br − ions to the surface during annealing at 80 °C after cleaving. Since we observe both Br − and Cl − ions as bright topographic features, the foremost atom in the tip apex must be Na + (ref. 35 ). High-resolution imaging of an isolated defect (insets in Fig. 1a ) shows that the corrugation amplitude of Br − is about three times larger than that of the Cl − ( Fig. 1b ), reflecting differences in their electronegativity, ionic radii and the position of Br − —predicted to be 20 pm above the surface plane by our calculations. The small topographic contrast between Cl and Br, being <0.1 nm, indicates that Br − ions are not adsorbed on the surface, but incorporated into the NaCl(001) surface layer, as substitutional species in the Cl − sublattice. Moreover, Br − ions showed remarkable stability as we could image them repeatedly in the same positions over the timescale of the experiment. Figure 1: Lateral atom manipulations. ( a ) Topography (left) and torsional frequency shift Δ f TR map (right) of the sodium chloride (NaCl) surface obtained at second flexural frequency shift Δ f 2nd =−144 Hz in an area of 28 × 28 nm, and ( b ) corresponding line profiles along A–A'. ( c ) Forward and backward topography maps, obtained at Δ f 2nd =−194 Hz in an area of 8.7 × 8.7 nm, revealing Br − manipulation events. ( d ) Models of three different types of manipulation deduced from the images in c . Measurement parameters for all images: amplitudes of the second flexural mode A 2nd =300 pm and the torsional mode A TR =50 pm. Full size image When scanning at smaller tip–sample separation, as in Fig. 1c , we observed different kinds of manipulation events for the Br − defects, following the processes pictured in Fig. 1d . These events are detected by sudden changes in the scanlines ( Supplementary Fig. 2 and Supplementary Note 2 ). The first event ( 1 in Fig. 1c ) appears as a lateral manipulation, exchanging Br − with a Cl − along the [100] direction. In the second event ( 2 in Fig. 1c ), Br − moves along the diagonal atomic row, and several more events of this type can be observed in the image. The third event ( 3 in Fig. 1c ) can be interpreted as a Br − moving from the non-imaged part of the surface, along the [110] or directions, or from the further site where it arrived after the second event, along the . Clearly, this lateral manipulation mechanism is more complicated compared with the case where an adatom laterally moves on top of the surface (standard lateral manipulation) [16] . Vertical atom manipulations In order to manipulate the Br − ions more controllably, we attempted manipulation by sequentially approaching the surface to pick up the ion, and approaching again to implant it back into the surface in the desired location. The procedure is equivalent to dynamic force spectroscopy. 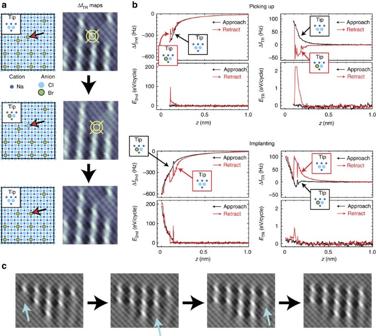Figure 2: Vertical atom manipulations. (a) ΔfTRmaps obtained before manipulation (top), after picking Br−(middle) and after implanting it back into the surface (bottom). Aside each image is the schematic view of the system. (b) Distance-dependent frequency shift and energy dissipation curves for both oscillation modes, measured while picking (top) and implanting (bottom) the Br−ion. Inset drawings show the tip apex during approach/retraction. (c) Series of ΔfTRmaps over an area of 6.4 × 5.1 nm showing the intermediate stages of an artificial ‘Swiss cross’ structure. Figure 2a (top) shows the Δ f TR maps at our starting point, with a schematic drawing of the atomic positions. During the imaging phase, the tip–sample distance needs to be sufficiently large to avoid accidental manipulations. The topographical contrast is then degraded and Δ f TR becomes the only means to accurately identify the atomic species. After imaging, we position the tip above the chosen Br − (marked in the image) and perform an approach-retraction sweep ( Fig. 2b ). We approach until the measured frequency shifts change abruptly, indicating a tip-change event as Br − was picked up. Figure 2: Vertical atom manipulations. ( a ) Δ f TR maps obtained before manipulation (top), after picking Br − (middle) and after implanting it back into the surface (bottom). Aside each image is the schematic view of the system. ( b ) Distance-dependent frequency shift and energy dissipation curves for both oscillation modes, measured while picking (top) and implanting (bottom) the Br − ion. Inset drawings show the tip apex during approach/retraction. ( c ) Series of Δ f TR maps over an area of 6.4 × 5.1 nm showing the intermediate stages of an artificial ‘Swiss cross’ structure. Full size image Subsequent imaging confirms that the target Br − ion has left the surface. The contrast before and after picking Br − remains the same, indicating that the apex atom is always a Na + , and the distortion caused by Br − in the tip is negligible ( Supplementary Note 2 ). The dissipation signals, on the other hand, increase with the doped tip, as the Br − defect makes its structure softer [36] , [37] . At this point we chose a target Cl − site on the surface (marked in Fig. 2a ; middle) and perform the implantation sweep, obtaining the signals shown in Fig. 2b (lower). During retraction we observe another tip-change event, suddenly decreasing Δ f 2nd and E 2nd , and subsequent imaging ( Fig. 2a ; lower) confirms that Br − was implanted in the desired position. The approach curves measured during pickup overlap with the retraction curves after implantation; the same is true for retraction after pickup and approach before implantation ( Supplementary Figs 3 and 4 and Supplementary Note 3 ). This indicates that the system switches reversibly between the two tip conditions, clean and Br − -doped. This remarkable stability enabled the procedure to be repeated several times, and as seen in Fig. 2c , during the whole experiment each pickup/implant process only manipulated the designated ion, leaving the others in their respective positions until completion of our design. Even though the process appears very controllable, the vertical manipulation must be a stochastic and rare event on the timescale of the oscillation cycle. If the jumps were happening on a smaller timescale, the dissipation signals would always be high because of the hysteresis in the forces [36] , [37] , yielding a high rate of failed depositions. This is not the case: dissipation is small and ~95% of the implantations are successful. The small amount of failed depositions is due to tip oscillating in the range of distances where pickup is more likely than implantation upon retraction, and re-pickup of Br − becomes possible. The implantation in Fig. 2b almost failed, leaving the trace of a double tip-change while retracting. Note that we believe, but cannot prove with the current model, that the re-pickup of Br − after implantation is usually prevented by a combination of factors: the different times spent in the pickup sensitive region during implantation and pickup; and changes in the tip apex structure after implantation. The experimental data reveal a remarkable statistical asymmetry between the two processes: implantation only occurs if the tip is approached 0.1 nm closer than the pickup sweep. This is a crucial aspect of the mechanism, allowing us to decide which event to trigger by tuning the approach distance of the cantilever. Theoretical calculations In order to understand the detailed process of the atomic manipulation, we performed theoretical calculations based on the density functional theory (DFT) of the manipulation mechanisms. The model system ( Fig. 3a ) includes an NaCl nanocluster tip and the NaCl surface with one substitutional Br − ion. The conventional lateral manipulation process [16] , involving the positional exchange of Br − with a neighbouring Cl − along the [110] direction, has a transition barrier of 1.9 eV, reduced to at most 1.5 eV by the presence of the tip ( Supplementary Fig. 5 and Supplementary Note 4 ). Although from visual inspection alone one might assume that all the processes in Fig. 1c could be the result of consecutive direct lateral manipulations, the energy barrier is too high and it is highly improbable that they could happen so often at RT. A more plausible model is that the tip effectively picks up Br − temporarily, allowing the vacancy underneath to diffuse, before the Br − drops to a new site. The barrier for vacancy diffusion is always low ( Supplementary Fig. 6 ), and proximity to the tip reduces the barrier for lifting Br − above the surface to the thermally active regime. Our calculations predict that this is impossible for the ideal tip shown in Fig. 3a , but the barrier becomes low enough if we consider a polar tip model ( Supplementary Fig. 7 )—a highly plausible tip model when measuring on insulators [38] , [39] , [40] , [41] . Our results show that the process is only viable at large tip-sample separation (>0.4 nm) and not directionally controlled, just as in experiments. Hence, we suggest this is the mechanism of apparent lateral manipulation seen in experiments. 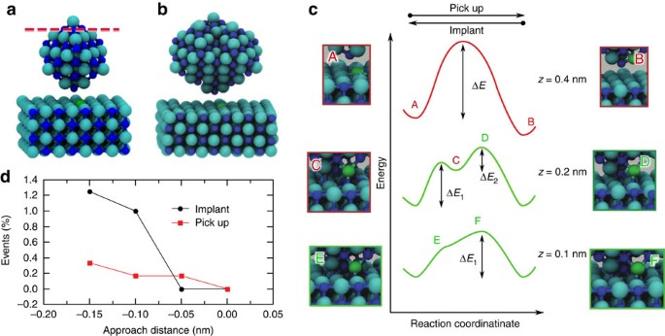Figure 3: Theoretical calculations. (a) Snapshot of the tip-surface system used in first principles calculations, with the dashed line marking the atoms removed to make a polar tip, and (b) classical simulations. Na+ions are dark blue, Cl−are cyan and Br−are green. (c) Schematic showing the development of the barrier as a function of tip-surface distance for the exchange of a substitutional Br−in the surface with a Cl−in the tip. (d) Statistical occurrence of implant and pickup events as a function of the tip-sample approach distance calculated from classical MD. Figure 3: Theoretical calculations. ( a ) Snapshot of the tip-surface system used in first principles calculations, with the dashed line marking the atoms removed to make a polar tip, and ( b ) classical simulations. Na + ions are dark blue, Cl − are cyan and Br − are green. ( c ) Schematic showing the development of the barrier as a function of tip-surface distance for the exchange of a substitutional Br − in the surface with a Cl − in the tip. ( d ) Statistical occurrence of implant and pickup events as a function of the tip-sample approach distance calculated from classical MD. Full size image We also performed similar calculations to study the possible exchange processes of Br − and Cl − intrinsic to the vertical manipulation (the analysis is equivalent when considering either the ideal or polar tip, see Supplementary Fig. 8 and Supplementary Note 5). The vertical process is approximated as the exchange of Br − on the surface, with a Cl − ion in the second atomic layer of the tip. This transition is called a pickup event, while the reverse process is labelled implantation. The approximation is consistent with the experimental observations as the tip apex atom never changes polarity as the manipulation is performed. Figure 3c shows a schematic of how the vertical manipulation barrier develops as a function of tip-surface distance. At a distance of 0.4 nm, there is a clear barrier (Δ E =1.5 eV) between the initial state with Br − in the surface A and the final state B with Br − at the tip. Note that B is lower in energy, as the system energetically prefers an ideal surface and Br − is less likely to return to the surface once attached to the tip. At a distance of 0.2 nm we see the appearance of two barriers, and a metastable state C with Br − bonded to both tip and surface. Picking up Br − requires overcoming a barrier of 0.8 eV to reach the metastable state C , and from there, jumping a smaller barrier of 0.2 eV to complete the process. In the opposite direction, the full barrier of 1.0 eV must be overcome to achieve implantation, making the process less likely (also see Supplementary Fig. 6 ). Hence, at this tip-surface distance picking up Br − becomes more likely than implanting it. Note that both events occur at smaller tip heights (<0.3 nm) than the regime for apparent lateral manipulation (>0.4 nm), showing a similar separation of manipulation processes to experiment. At closer approach (0.1 nm or below), the metastable position disappears and the single barrier (Δ E 1 ) is ~0.8 eV, making both transitions equally possible at RT. Below this separation, DFT methods suffer from convergence problems, as too many transition paths become available, therefore we performed RT classical molecular dynamics (MD) simulations to study the complex configurations in this regime ( Supplementary Note 4 ). Two model systems were built ( Fig. 3b ), representing the stable configurations A and B . We then simulated the vertical oscillation of the tip, and observed whether a pickup or implantation event occurred depending on the final position of the Br − ion. By repeating the simulation 400 times for each approach distance, with different initial conditions, we calculated the occurrence probability of configuration jumps, shown in Fig. 3d . In all simulated cycles, we never observed a direct lateral manipulation event, confirming the prediction from DFT calculations. The results indicate how implantation becomes more dominant than pickup at closer approach—the different regimes are separated by ~0.05–0.10 nm, compared with 0.1 nm in experiments (but also see discussion in Methods). Both processes are actually rare for a given oscillation cycle: theory and experiment agree well on this point. Complex pattern in the NaCl(001) surface Finally, the vertical manipulation was successfully performed several times, perfectly aligning 20 Br − ions in the NaCl surface, forming a ‘Swiss cross’ with a size of 5.64 × 5.64 nm ( Fig. 4 and Supplementary Movie 1 ). Note that this is the largest number of the atomic manipulations ever achieved at RT. The Br − ions are positioned at every other Cl − ion site on the surface, and the fabricated cross is stable for a relatively long time (see Supplementary Fig. 9 ). 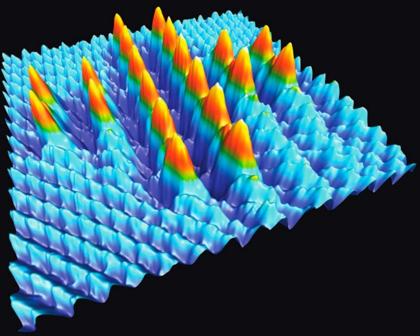Figure 4: ΔfTRmap of the completed ‘Swiss cross’ structure obtained through manipulation of Br−ions. The size of the cross is 5.64 × 5.64 nm and contains 20 Br−ions. Figure 4: Δ f TR map of the completed ‘Swiss cross’ structure obtained through manipulation of Br − ions. The size of the cross is 5.64 × 5.64 nm and contains 20 Br − ions. Full size image In conclusion, by combining bimodal dynamic force microscopy and theoretical methods, we were able to identify the two manipulation mechanisms of Br − impurities in the NaCl(001) surface—apparent lateral manipulation via the transitory pickup of Br − and vertical manipulation via exchange of Br − in surface and Cl − in the tip. For vertical manipulation, the statistical asymmetry between picking and implanting transitions allowed the possibility of controllably manipulating Br − ions from and to chosen positions, in contrast to the more random lateral manipulation process. Ultimately, we designed the ‘Swiss cross’ with 20 Br − ions on the NaCl(001) surface as a benchmark case of atomic manipulation on an insulating surface at RT. This work, together with previous studies on metals and semiconductors, shows how systematic atomic manipulation at RT, on any class of surface, is now possible. This is an important step towards the fabrication of advanced electromechanical systems at the nanoscale, in a bottom–up manner. Experimental measurement All experiments were performed with home-made AFM with a silicon cantilever [42] , operating at RT in UHV. A NaCl crystal was cleaved in UHV to present the (001) surface. Subsequently, it was annealed at 80 ° C for several hours to remove the charges caused by in situ UHV cleaving. The thickness of the sample was ~5 mm. A commercially available Si cantilever (Nanosensor NCL-PPP) was used as a force sensor. It was annealed at 150 °C and subsequently the tip was cleaned by Ar + sputtering (680 eV for 90 s). Before the measurements, the tip was gently contacted to the sample surface, and so that the tip apex was assumed to be covered with the sample material of NaCl (ref. 43 ). Our measurements were performed in bimodal operation mode [33] ( Supplementary Fig. 10 ), using the second flexural [44] , [45] , [46] and first torsional resonance modes [48] , [47] to oscillate the tip apex vertically and laterally with respect to the sample surface, respectively. These frequency shifts were detected with two sets of a digital phase-locked loop (Nanonis: dual-OC4). The second flexural mode was chosen because its high effective stiffness k 2nd =1,548 N m −1 enables stable measurements of the vertical tip–sample interaction with small amplitudes, enhancing sensitivity to normal forces [49] . The torsional dithering of the tip was mainly along the fast-scan X direction, effectively measuring the lateral force gradient as F ′ X =−2 k TR Δ f TR / f TR , where k TR is the stiffness of the torsional mode, f TR the torsional resonance frequency and Δ f TR the frequency shift [50] . The stiffness of the torsional mode was calculated from the dimensions of the cantilever and its material properties. The parameters of the cantilever are listed in Supplementary Table 2 . Given the small vertical oscillation amplitude of 300 pm, the contribution of the site-independent electrostatic force between the sharp Si tip and the sample surface is negligible, therefore it was not necessary to compensate for it with an external bias voltage. The bias voltage between the tip and the surface was always set to 0 V. Measured images were analysed using the WSxM software [51] . In the small Z range of 0.21–0.23 nm ( Fig. 2b ), the driving voltage to the torsional oscillation is saturated even by a tiny tip–sample dissipative interaction of 2.2 meV per cycle and hence the oscillation amplitude is reduced. This is due to the fact that a finite dynamic range of the PLL output restricts a magnitude of the controllable damping, which essentially becomes difficult to be controlled using an oscillation mode with such an ultra small intrinsic loss of oscillation (0.79 μeV per cycle), a high mechanical quality factor of 12,4385 and an ultra small amplitude of 50 pm. Nevertheless, unlike the vertical oscillation, the reduction of the torsional amplitude affects the tip–sample interaction much less because the oscillation amplitude is already small enough to detect the force gradient directly. Theoretical calculation All first-principles calculations in this work were performed using periodic plane–wave basis VASP code [52] , [53] , implementing the spin-polarized DFT and the generalized gradient approximation. Projected augmented wave potentials [54] , [55] were used to describe the core electrons. A kinetic energy cutoff of 280 eV was found to converge the total energy of the tip-surface systems to within 10 meV. Systematic k-point convergence was checked for smaller bulk and surface calculations, but for the large surface unit cell used in the NC-AFM simulations the gamma point was sufficient to converge energies and forces to a high tolerance. All atomic forces were minimised to a tolerance of 0.02 eV Å −1 . All diffusion barriers were determined using the climbing image nudged elastic band method [56] . To model the NaCl surface, we used a 4 × 4 × 2 slab in terms of the NaCl unit cell, infinitely repeated in x and y , with a vacuum gap of over 1 nm in z . The bottom two layers were kept frozen to represent the macroscopic sample, while all other atoms were allowed to relax. As discussed in the text of Fig. 1a , it is clear that the tip must be positively terminated to image Br − impurities as bright [57] . Furthermore, there is no evidence of atomic chain formation [36] , so the nanotip must be relatively stable during scanning. Hence, we chose as a tip model an ideal Na 32 Cl 32 cube, oriented with one Na + ion at the lower apex closest to the surface ( Fig. 3a ). The assumption of contamination of the originally oxidized silicon tip by surface material is standard in AFM studies of insulators [35] . In order to represent the macroscopic part of the tip, the upper third of the tip was kept frozen while all other atoms were allowed to relax. The polar tip model was created by removing the top two atomic layers from the tip (marked by the dashed line in Fig. 3a in the main paper), producing an excess of Cl − ions at the tip of the top and a dipole of ~5 e (24 D) in the z direction. The MD calculations applied a classical model treating atoms as massive point charges interacting through electrostatic and short-range empirical potentials [58] . The physical properties of the considered species are listed in Supplementary Table 3 . The total potential energy of the system is given by: where q i are the ion charges, r ij is the distance between ionic pairs and A ij , B ij and ρ ij are parameters defined for each type of ionic pair. The first term gives the long-range electrostatic interaction, and the second one represents the short-range Buckingham type interaction [58] : parameters for all ionic pairs were obtained from previous studies [59] , [60] , [61] and are listed in Supplementary Table 4 . It should be mentioned that the short-range interaction between two Br − ions is neglected since only one Br − ion is present in the simulation at any time. The ideal surface is represented by a slab consisting of 10 × 10 × 4 NaCl atoms; from this, the Br − doped surface is obtained by replacing the central Cl − ion in the surface layer with a Br − ion. Owing to the finite size of the simulation, that is, no periodic boundary conditions are enforced, the atoms in the boundary of the slab are harmonically restrained around their ideal positions and coupled to a thermostat. The tip is modelled starting from an ideal Na 32 Cl 32 cube (as in the DFT model), from which the three upper surfaces were extended by another two 4 × 4 atomic layers. Atoms in these additional layers are tethered to virtual points, located in their ideal initial positions, and their velocities are coupled to a second thermostat. The extended cube model is necessary in dynamical simulations as the symmetry of restrained part must respect the symmetry of the rest of the tip: the lack of such consideration induces artificial oscillations of the apex. Both tip and surface thermostats are set to 300 K, and all the non-tethered atoms are treated as newtonian. Starting from these models, we build two different configurations: in one case a substitutional Br − impurity sits in the surface and the tip is clean NaCl, while in the other, the Br − is found in the second atomic layer of the apex and the surface is ideal. We place the tip so that the Br − impurity in its second atomic layer is located above a surface Cl − ion, in order to facilitate the transition; the vertical separation is measured by the initial distance between the tip foremost atom and the surface plane. The flexural oscillation of the NC-AFM tip can be imposed by displacing the tether points along an harmonic trajectory, with a frequency of 150 MHz: this is chosen higher than the experimental value for computational efficiency, but still several orders of magnitude slower than the atomic vibrational frequency and was found not to alter the results. We set the oscillation amplitude to 1 nm, although only a downward portion of the whole cycle is simulated, sweeping across a vertical distance of 0.7 nm. By tracking the position of the Br − ion it becomes possible to observe whether it jumps from/onto the tip and repeating the cycle 400 times ensures a good statistical sample. The simulation is repeated using different initial tip–surface separation for both systems, ultimately giving the jump probability as a function of distance. As in experiments, we observe a slight shift of the active deposition site compared with the pickup site. It is important to note that the tip–surface distance scales of the manipulation processes must be carefully compared between the DFT and classical models. On the timescale of experiments (minutes), we know that a barrier of 0.5 eV could be thermally activated, but this is far beyond the timescale of the MD simulations (nanoseconds). This means that we cannot be sure that the jump crossover (pickup/implantation) seen in the MD would not be seen at larger distances than the −0.05 nm predicted, but the DFT provides a strong upper limit of 0.05 nm. How to cite this article: Kawai, S. et al. Atom manipulation on an insulating surface at room temperature. Nat. Commun. 5:4403 doi: 10.1038/ncomms5403 (2014).